Characterising side chains in large proteins by protonless13C-detected NMR spectroscopy Side chains cover protein surfaces and are fundamental to processes as diverse as substrate recognition, protein folding and enzyme catalysis. However, characterisation of side-chain motions has so far been restricted to small proteins and methyl-bearing side chains. Here we present a class of methods, based on 13 C-detected NMR spectroscopy, to more generally quantify motions and interactions of side chains in medium-to-large proteins. A single, uniformly isotopically labelled sample is sufficient to characterise the side chains of six different amino acid types. Side-chain conformational dynamics on the millisecond time-scale can be quantified by incorporating chemical exchange saturation transfer (CEST) into the presented methods, whilst long-range 13 C- 13 C scalar couplings reporting on nanosecond to millisecond motions can be quantified in proteins as large as 80 kDa. The presented class of methods promises characterisation of side-chain behaviour at a level that has so far been reserved for the protein backbone. Proteins are dynamic entities whose molecular function is intrinsically related to their structure and dynamic sampling, both in the immediate vicinity of active sites and in regulatory sites [1] , [2] . Proteins are often viewed as representations of their backbone and most experimental studies of protein dynamics to date have primarily focussed on the protein backbone, with much less attention paid to side chains [3] , [4] , [5] , [6] , [7] , [8] , [9] . Whilst knowledge of the behaviour of the protein backbone is essential in order to understand many aspects of protein function, bringing side chains into focus is crucial. It is the side chains that give the amino acids in proteins their unique chemical diversity, for example, side chains form critical parts of many active sites of enzymes and the side chains presented on the protein surface are key to substrate recognition and binding events. In many cases, the dynamics and interactions of side chains are as, if not more, important to the biological function than the overall backbone conformation. In addition, the motions of side chains are often decorrelated from the backbone [10] , [11] , [12] . In order to understand the mechanisms of enzymes and characterise macromolecular interactions and regulation, it is imperative to be able to specifically characterise the side-chain structure and movements. Nuclear magnetic resonance (NMR) spectroscopy is uniquely situated to generally characterise the interactions and conformational sampling of side chains in proteins. However, most experimental studies of protein motions using NMR spectroscopy to date have focussed on the backbone or methyl groups, and detailed information regarding side-chain behaviour has been restricted to small proteins [13] , [14] and methyl-bearing side chains [15] , [16] , [17] . The limitations of currently available approaches are mainly due to line broadening and signal loss as a result of efficient relaxation pathways, as well as insufficient resolution and signal overlap in the NMR correlation maps used to extract parameters reporting on dynamics and interactions. Here, we present a class of NMR methods that allows a more general characterisation of side chains in medium-to-large proteins. The presented class of methods is anchored in 13 C-direct detection [18] NMR spectroscopy of per-deuterated proteins. The slow relaxation of the aliphatic 13 C nuclei in deuterated proteins results in sharp NMR signals, whilst the correlation of two 13 C chemical shifts results in high-resolution and well-resolved two-dimensional NMR spectra. It is shown that the slow transverse 13 C relaxation rates enable a large range of NMR experiments to be performed to characterise the structure, interactions and dynamics of side chains in medium-to-large (< 82 kDa) proteins. The presented experiments include a quantification of long-range 13 C– 13 C scalar couplings [13] reporting on the sampling of side-chain dihedral angles and chemical exchange saturation transfer (CEST) experiments [19] to characterise low-populated states. Side-chain 13 C– 13 C correlation spectra The BMRB [20] databank provides a large database of assigned NMR chemical shifts, including the side-chain 13 C chemical shift. Analysis of these data reveals six side chains (Fig. 1; Supplementary Fig. 1) with a ‘terminal’ 13 C ( 13 C t ), which is directly bonded to just one other 13 C and which has a chemical shift distribution that is isolated from its directly bonded penultimate 13 C ( 13 C p ). This distinct chemical shift profile means that the terminal 13 C t can be selectively excited in an NMR experiment using frequency-selective pulses. Selective excitation enables spectral filtering and observation of specific residue types in multidimensional NMR spectra, even when using uniformly isotopically labelled proteins. Fig. 1 Examples of aliphatic 13 C chemical shift distributions. Distribution of the assigned 13 C chemical shifts of ( a ) arginine and isoleucine ( b ) residues extracted from the BMRB [20] databank. Terminal 13 C t , directly coupled to just one other 13 C are coloured blue and the bonded, penultimate 13 C p , are  coloured red. For clarity, only one of the two 13 C t – 13 C p pairs have been highlighted in isoleucine (See Supplementary Fig. 1 for other sites) Full size image The core element of the presented side-chain-specific NMR experiments, Fig. 2a , correlates the terminal carbon 13 C t with its directly bonded penultimate 13 C p within a protein side chain. The terminal 13 C t includes 13 C δ in the arginine side chains, 13 C δ1 and 13 C γ2 in isoleucine, 13 C ε in lysine, 13 C δ in proline, 13 C γ2 in threonine and 13 C γ in valine residues. The fact that the magnetisation of interest starts and is detected on the terminal 13 C t has some key advantages. The homonuclear coupling pattern for 13 C t is a simple doublet, which allows for the magnetisation of interest to be transferred completely between 13 C t and 13 C p using simple INEPTs and also facilitates virtual decoupling in the 13 C t detected dimension. Fig. 2 13 C– 13 C side-chain correlation spectra of per-deuterated proteins. a Schematic representation of the NMR pulse sequence used to obtain 13 C– 13 C side-chain correlation spectra. The flow of the magnetisation between 13 C t (blue) and 13 C p (red) is shown above the sequence with colour gradients. The following delays are used: Δ = 1/(4 J CC ) ≈ 7.1 ms, T = 1/(2 J CC ) ≈ 14.1 ms, where J CC is the one-bond 13 C– 13 C scalar coupling constant. Rectangular pulses are high-power and not selective, bell-shaped pulses are frequency selective (90°: white outlined, 180°: black). Deuterium, 2 H, is decoupled throughout the sequence and frequency discrimination is obtained by states–TPPI of phase ϕ [21] . b Schematic representation of post-processing to obtain the decoupled spectrum. c Arginine 13 C δ – 13 C γ correlation of the 18-kDa protein T4L L99A, obtained on a 1.4 mM sample at a static field of 14.1 T at 278 K in 37 min Full size image In the core experiment, Fig. 2a and Supplementary Fig. 2 , magnetisation is initially transferred from 13 C t to 13 C p , then labelled with the chemical shift of 13 C p during t 1 and finally transferred back to 13 C t for detection. The doublet peak splitting observed for 13 C t because of the evolution of the single one-bond 13 C t – 13 C p scalar coupling during acquisition ( t 2 ) can conveniently be resolved by recording two sub-spectra, in-phase (IP) and anti-phase (AP) [22] . Figure 2b shows how subsequent post-processing is used to virtually ‘decouple’ the spectra in the direct 13 C t dimension, so that single peaks are observed in multidimensional correlation spectra. 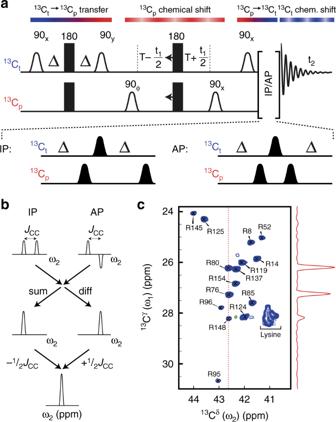Fig. 2 13C–13C side-chain correlation spectra of per-deuterated proteins.aSchematic representation of the NMR pulse sequence used to obtain13C–13C side-chain correlation spectra. The flow of the magnetisation between13Ct(blue) and13Cp(red) is shown above the sequence with colour gradients. The following delays are used: Δ = 1/(4JCC) ≈ 7.1 ms, T = 1/(2JCC) ≈ 14.1 ms, whereJCCis the one-bond13C–13C scalar coupling constant. Rectangular pulses are high-power and not selective, bell-shaped pulses are frequency selective (90°: white outlined, 180°: black). Deuterium,2H, is decoupled throughout the sequence and frequency discrimination is obtained by states–TPPI of phase ϕ21.bSchematic representation of post-processing to obtain the decoupled spectrum.cArginine13Cδ–13Cγcorrelation of the 18-kDa protein T4L L99A, obtained on a 1.4 mM sample at a static field of 14.1 T at 278 K in 37 min One-bond 13 C– 13 C couplings in indirect dimensions ( t 1 ) are removed using constant-time evolutions [23] , and evolutions of the 2 H– 13 C couplings are efficiently suppressed using 2 H decoupling (see Supplementary Fig. 2 ). Application of the method to observe 13 C– 13 C correlations in the 18-kDa L99A mutant of T4 lysozyme (T4L L99A) is shown for arginine 13 C δ – 13 C γ in Fig. 2c, and for other side-chain correlations in Supplementary Figs. 3 and 4 . Of importance is that (1) the NMR correlation spectrum in Fig. 2c is obtained in 37 min at 278 K, where the rotational correlation time of the 18-kDa T4L L99A mimics that of an ~30-kDa protein at room temperature, (2) six different 13 C– 13 C correlation maps can be obtained in less than 12 min (see Supplementary Figs. 3, 4 ) and (3) a single uniformly [ 2 H, 13 C] isotopically labelled sample could be used to characterise six side chains. 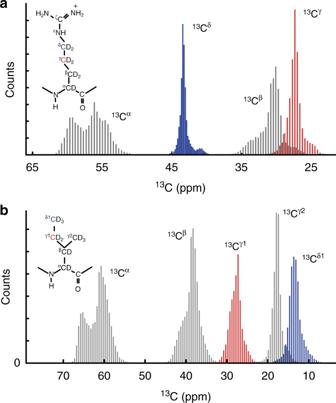The lack of directly bonded protons and absence of efficient relaxation pathways for aliphatic 13 C in highly deuterated proteins dramatically reduces the 13 C relaxation rates. Fig. 1 Examples of aliphatic13C chemical shift distributions. Distribution of the assigned13C chemical shifts of (a) arginine and isoleucine (b) residues extracted from the BMRB20databank. Terminal13Ct, directly coupled to just one other13C are coloured blue and the bonded, penultimate13Cp, are  coloured red. For clarity, only one of the two13Ct–13Cppairs have been highlighted in isoleucine (See Supplementary Fig.1for other sites) For T4L L99A, the isoleucine 13 C δ1 non-selective longitudinal relaxation rates, R 1 , range between 0.12 and 0.24 s −1 at 278 K and a field of 14.1 T (see Supplementary Table 1 and Supplementary Fig. 5) . This necessitates longer recycling delays and fewer scans per unit time, and the lower gyromagnetic ratio of 13 C compared with 1 H leads to an intrinsic lower signal-to-noise. However, reduced relaxation rates also lead to small transverse relaxation rates, between 2.7 and 8.8 s −1 for isoleucine 13 C δ1 in T4L L99A at 278 K and 14.1 T (see Supplementary Table 2 and Supplementary Fig. 7 ), which in turn lead to very sharp signals. For example, with the 13 C-detected method, it became possible to observe sites in arginine side chains of T4L L99A that were not detectable in a 1 H-detected equivalent experiment, even when using a highly optimised isotope-labelling scheme (Supplementary Fig. 6 ). Another striking advantage of 13 C– 13 C correlation spectra compared with 1 H– 13 C spectra is the substantially better chemical shift dispersion in the directly detected dimension, resulting in significantly better peak separation (see Supplementary Fig. 6 for a comparison). Moreover, as compared with 1 H– 13 C spectra, the 13 C– 13 C correlation maps directly provide the chemical shift of two aliphatic 13 C that are both known to report on the structure and sampling of side chains [24] , [25] . Direct-detected 13 C spectra of a 82-kDa protein The excellent spectra obtained on the medium-sized T4L L99A protein at low temperature and the favourable 13 C transverse relaxation rates show that 13 C-direct detection is ideally suited for characterising side chains in large proteins. Side-chain 13 C– 13 C correlation maps were recorded for the significantly larger 82-kDa malate synthase G (MSG) protein [26] . 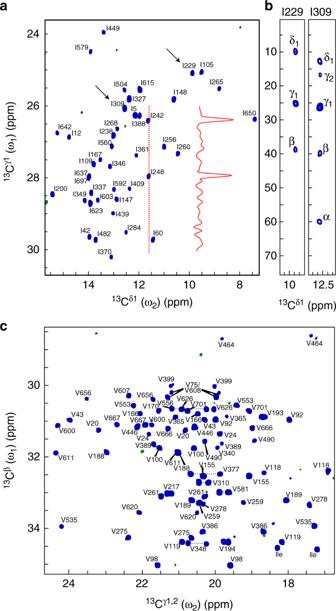Fig. 3 13C–13C side-chain correlation spectra of a large protein.aIsoleucine13Cδ1–13Cγ1andcvaline13Cγ–13Cβcorrelation spectra of a 0.5 mM sample of the 82-kDa protein MSG. Each of the two spectra inaandcwere recorded in 7.5 h at 18.8 T using a standard helium-cooled Bruker TCI radio-frequency probe.bCorrelating the13Cδ1–13Cγ1of isoleucine with the rest of the side chain13C for chemical shift assignment. Representative TOCSY strips from a three-dimensional13C-detected CC-TOCSY experiment (see Supplementary Fig.8) for I229 and I309 (marked with black arrows ina. Chemical shift assignments inaandcwere obtained from (refs.26,27) combined with the 3D-CC-TOCSY. Peaks labelled Ile incare isoleucine13Cγ2–13Cβcorrelations. All experimental parameters are given in Supplementary Materials and Methods Figure 3a and c shows the isoleucine 13 C δ1 – 13 C γ1 and valine 13 C γ – 13 C β correlation maps of MSG, respectively, where excellent chemical shift dispersion and resolution result in nearly no overlap of peaks even in this large and uniformly [ 2 H, 13 C] isotopically labelled system. The slow transverse relaxation rate of aliphatic 13 C in per-deuterated proteins means that the experiment shown in Fig. 2a easily can be extended to obtain numerous other NMR parameters reporting on motions, conformations and interactions. TOtal Correlated SpectroscopY (TOCSY) NMR experiments are typically used to aid side-chain chemical shift assignment [28] of proteins and a couple of representative examples are shown in Fig. 3b for MSG, with details of the sequence given in Supplementary Fig. 8 . Fig. 3 13 C– 13 C side-chain correlation spectra of a large protein. a Isoleucine 13 C δ1 – 13 C γ1 and c valine 13 C γ – 13 C β correlation spectra of a 0.5 mM sample of the 82-kDa protein MSG. Each of the two spectra in a and c were recorded in 7.5 h at 18.8 T using a standard helium-cooled Bruker TCI radio-frequency probe. b Correlating the 13 C δ1 – 13 C γ1 of isoleucine with the rest of the side chain 13 C for chemical shift assignment. Representative TOCSY strips from a three-dimensional 13 C-detected CC-TOCSY experiment (see Supplementary Fig. 8 ) for I229 and I309 (marked with black arrows in a . Chemical shift assignments in a and c were obtained from (refs. [26] , [27] ) combined with the 3D-CC-TOCSY. Peaks labelled Ile in c are isoleucine 13 C γ2 – 13 C β correlations. All experimental parameters are given in Supplementary Materials and Methods Full size image Characterisation of millisecond dynamics A full characterisation of the role of side chains requires an appreciation of their motions within the protein. Of substantial importance is that the method detailed above can be extended to allow quantification of side-chain motions across a wide range of timescales. Although many experiments will be possible using the new scheme, two examples, which together report on side-chain motions on timescales from nanoseconds to milliseconds, were chosen here to highlight the versatile applicability. Protein dynamics and conformational exchange on the millisecond timescale have been shown to be important for the function of many proteins [29] and the chemical exchange saturation transfers (CEST) [19] , [30] NMR experiment, amongst others, allows a quantification of exchange events on this timescale. CEST experiments have recently been adapted for side chains in small proteins [14] , in a 1 H-detected manner. Integrating CEST with the 13 C-detected method described above (see Supplementary Fig. 9 ) allows quantification of side-chain conformational exchange in medium-to-large proteins between the ground state (G) and an excited state (E). Examples of CEST profiles are shown in Fig. 4 and Supplementary Fig. 9 , where the conformational exchange of T4L L99A at 278 K is quantified by a 13 C-detected CEST experiment. The calculated overall exchange rate, k ex = 128 ± 18 s −1 , and the population of the excited state, p E = 1.15 ± 0.11% (see Supplementary Fig. 10 ), agree well with previous studies [11] showing that reliable parameters are derived from 13 C-detected CEST experiments. The chemical shifts of aliphatic 13 C within the protein side chains report on the rotameric sampling of the side chain [24] , and the results of the CEST experiments in Fig. 4 also report on the rotameric sampling in the excited state. Specifically, from the chemical shifts obtained for V103 in the ground and excited states, ϖ G and ϖ E , respectively, it can be calculated [24] that the χ 1 angle of V103 changes from a predominantly trans conformation (91% trans, 9% gauche-plus) in the ground state to a mainly gauche-minus conformation in the excited state (26% gauche-plus, 16% trans, 58% gauche-minus), which is in agreement with the existing structures of T4L L99A in the ground and the excited state [11] . Access to the 13 C chemical shifts in the excited state via the 13 C-detected CEST experiment also reveals that the V103 side chain is more dynamic in the excited state with a broader distribution of side-chain rotamers. Fig. 4 Quantifying side-chain motions on the millisecond timescale. CEST profiles to quantify millisecond chemical exchange of V103 13 C γ2 in T4L L99A at 278 K are shown. The circles represent experimentally obtained normalised intensities, and the lines are the result of a least-squares fit. Uncertainties in the reported ϖ G and ϖ E are obtained using the covariance method in the least-squares fit (see Materials and Methods for full details) Full size image Measuring long-range 13 C– 13 C scalar couplings The second application involves the measurement of three-bond 13 C δ – 13 C α scalar couplings [13] , 3 J CαCδ , reporting on the conformational sampling of the side-chain χ 2 dihedral angle on a timescale from nanoseconds to milliseconds. The three-bond scalar coupling 3 J CαCδ relates to the side-chain χ 2 dihedral angle via a Karplus relationship, where large coupling constants are observed when the χ 2 angle is in a trans conformation, and small couplings are observed when χ 2 is in a gauche conformation. Intermediate values of the coupling constant are observed when the side chain is dynamic about the χ 2 dihedral angle. Extending the 13 C– 13 C correlation experiment to measure these couplings (see Supplementary Fig. 10 ) showed that the majority of the arginine side chains in T4L L99A are predominantly in a trans conformation around the χ 2 angle (see Supplementary Table 3 ) in agreement with crystallographic data. For the two arginine side chains of T4L L99A shown in Fig. 5a , the intermediate value of the coupling constant for R14 shows that this side chain is flexible and dynamic around the χ 2 angle, while the high value observed for the R148 side chain shows a rigid trans conformation. This is in good agreement with previous characterisations of the dynamics of the arginine side chains of T4L L99A [6] , [31] , [32] , as well as with the structure of T4L L99A, where R14 is on the surface and R148 is engaged in a salt bridge with D10. Long-range 13 C δ – 13 C α scalar couplings were also measured for isoleucine residues in the 82 -kDa MSG protein (Fig. 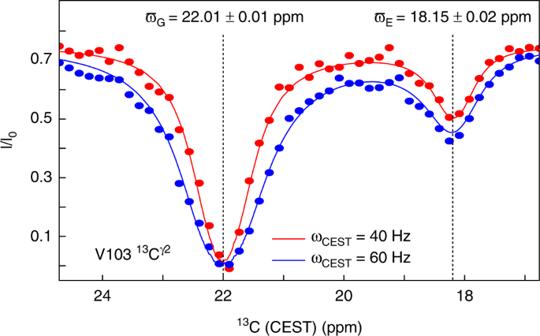Fig. 4 Quantifying side-chain motions on the millisecond timescale. CEST profiles to quantify millisecond chemical exchange of V10313Cγ2in T4L L99A at 278 K are shown. The circles represent experimentally obtained normalised intensities, and the lines are the result of a least-squares fit. Uncertainties in the reportedϖGandϖEare obtained using the covariance method in the least-squares fit (see Materials and Methods for full details) 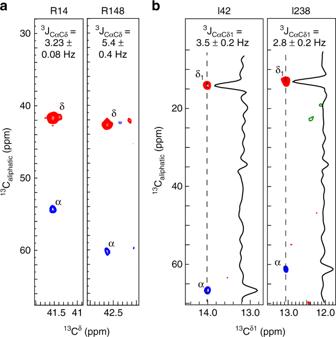Fig. 5 Quantifying long-range scalar13C–13C couplings.aTwo examples of strips used to quantify long-range13Cδ–13Cαscalar couplings in the arginine side chains of T4L L99A at 18.8 T and 278 K. The R14 side chain is flexible, while the R148 is rigid in agreement with relaxation measurements6.bStrips from a three-dimensional experiment to quantify long-range13Cδ1–13Cαscalar couplings in isoleucine side chains of the 82-kDa MSG at 14.1 T and 310 K. The I238 side chain is dynamic around the χ2angle, as seen by the intermediate value of the3JCαCδ1coupling constant, whereas I42 is more rigid in a trans conformation. Positive contours are depicted as red, while negative contours are in blue. Values for3JCαCδ1inaandbare mean ± s.d. 5b ; Supplementary Table 4 ). Of the 44 isoleucine residues in MSG, 13 C δ – 13 C α scalar couplings were obtained for 32, allowing a quantification of the dynamics of these side chains. Access to both the 13 C δ1 chemical shift and the 13 C δ1 – 13 C α scalar coupling allows a full characterisation of the rotameric sampling about the χ 2 angle. For example, a large 13 C δ1 chemical shift and a small 13 C δ1 – 13 C α coupling for I200 in MSG show that this residue is restrained in a rare gauche-plus state (see Supplementary Table 4 ) [25] , in agreement with the crystal structure of MSG. Fig. 5 Quantifying long-range scalar 13 C– 13 C couplings. a Two examples of strips used to quantify long-range 13 C δ – 13 C α scalar couplings in the arginine side chains of T4L L99A at 18.8 T and 278 K. The R14 side chain is flexible, while the R148 is rigid in agreement with relaxation measurements [6] . b Strips from a three-dimensional experiment to quantify long-range 13 C δ1 – 13 C α scalar couplings in isoleucine side chains of the 82-kDa MSG at 14.1 T and 310 K. The I238 side chain is dynamic around the χ 2 angle, as seen by the intermediate value of the 3 J CαCδ1 coupling constant, whereas I42 is more rigid in a trans conformation. Positive contours are depicted as red, while negative contours are in blue. Values for 3 J CαCδ1 in a and b are mean ± s.d. Full size image A strategy to characterise side chains in proteins using 13 C-direct-detected NMR has been developed. Applications of 13 C-detection to macromolecules has so far mainly been employed to investigate intrinsically disordered regions [18] , [22] , where many experiments are now available to exploit the improved resolution of 13 C compared with 1 H. Existing methods to characterise side chains in medium-to-large proteins have been limited to methyl-bearing residues and require specific labelling. The presented method employs 13 C-detection and capitalises on the distinct chemical shift profiles of side chains to specifically observe different residues in a single uniformly labelled sample. As such, it allows a more general characterisation of side chains for investigations in large proteins (~82 kDa) and for a quantification of the dynamics of these side chains. The slow transverse 13 C relaxations rates in fully deuterated proteins enables a large range of NMR experiments to characterise side-chain structure, interactions and dynamics. A few examples of experiments integrated with the side-chain 13 C– 13 C-direct-detected method are detailed above. Combined with recent developments of hardware aimed at 13 C-direct-detected NMR spectroscopy, we envisage that the new method will be particularly useful for experimentally quantifying functional side chains, at atomic resolution, in medium-to-large proteins. Forthcoming applications of this suite of methods promise a burgeoning appreciation of the role side chains play in orchestrating protein function. Sample preparations Isotopically labelled T4 lysozyme mutant C54T/C97A/L99A (T4L L99A) was expressed and purified as described previously [33] . Briefly, a codon-optimised form of the gene containing the mutations L99A, C54A and C97A in a kanamycin-resistant, pET-29b vector was transformed into BL21 (DE3) chemically competent E. coli cells. A single colony was used to inoculate 5-mL culture, which was grown overnight at 37 °C. This was used to inoculate 50 mL of minimal M9 media made with 2 H 2 O and supplemented with 1 g L −1 [ 1 H, 15 N]-ammonium chloride as the sole nitrogen source. For the uniformly labelled [ 2 H, 13 C, 15 N] sample, 2 g L −1 [ 2 H, 13 C]-glucose was added as the sole carbon source. For the [ 1 H 13 C-Lys,Arg; 2 H 12 C] isotopically labelled sample, 2 g L −1 [ 2 H, 12 C]-glucose was added to the media, and 0.15 g L −1 [ 1 H 13 C]-L-lysine, and 0.15 g L −1 [ 1 H, 13 C]-L-arginine was later added 1 h prior to induction. This culture was grown overnight at 37 °C and used to inoculate a final 2-L culture. The final culture was grown to OD 600 ≈ 0.6 before a 16-h induction with 1 mM IPTG at 18 °C. The T4L L99A protein was initially purified by ion-exchange chromatography. After lysis by sonication in (50 mM NaPO 4 (pH 6.5), 2 mM EDTA, 5 mg of DNAse1 (Sigma) and 1 cOmplete TM Mini Protease Inhibitor Cocktail tablet (Sigma) per 50-mL lysate), the soluble fraction was loaded onto a 5-mL HiTrap SP Sepharose FF column (GE Healthcare) (50 mM NaPO 4 (pH 6.5), 2 mM EDTA). Protein was eluted from the column using a gradient of 1 M NaCl and T4L99A eluted at ~300 mM NaCl. Pooled fractions were further purified by size-exclusion chromatography using a Superdex S75 gel filtration column (GE Healthcare) (50 mM NaPO 4 (pH 5.5), 2 mM EDTA and 25 mM NaCl). Pooled fractions were buffer exchanged into the final NMR buffer (50 mM NaPO 4 (pH 5.5), 2 mM EDTA, 25 mM NaCl and 2 mM NaN 3 ). The NMR sample contained 1.4 mM protein in 95%/5% 1 H 2 O/ 2 H 2 O for the uniformly [ 2 H 13 C 15 N] labelled sample and 1.5 mM protein in 100% 2 H 2 O for the [ 1 H 13 C-Lys,Arg; 2 H 12 C] labelled sample. Isotopically labelled MSG was produced as described previously [26] . The gene with a C-terminal hexahistidine tag in an kanamycin-resistant pET-28a vector was transformed into BL21 (DE3) chemically competent E. coli cells. A single colony was used to inoculate 5-mL culture, which was grown overnight at 37 °C. This was used to inoculate 50 mL of M9 minimal media made with 2 H 2 O and supplemented with 1 g L −1 [ 1 H, 15 N]-ammonium chloride and 2 g L −1 of [ 2 H, 13 C]-glucose as the sole nitrogen and carbon sources, respectively. The pre-culture was used to inoculate 1 L of M9 media, which was grown at 37 °C to OD 600 ≈0.45 before a 1-in-2 dilution to make the final 2-L culture volume. This final culture was grown to OD 600 ≈ 0.45 before a > 16-h induction with 1 mM IPTG at 16 °C. The MSG protein was initially purified by affinity chromatography. After lysis by sonication (20 mM Tris, 300 mM NaCl, 20 mM 2-mercaptoethanol, 10 mg of DNase1 (Sigma), 10 mg of hen egg lysozyme (Sigma) and 1 cOmplete TM Mini Protease Inhibitor Cocktail tablet (Sigma) per 50-mL lysate), the soluble fraction was loaded onto a HisTrap 5-mL HP column (GE Healthcare) (20 mM Tris, 300 mM NaCl and 20 mM 2-mercaptoethanol, pH 7.8). Protein was eluted from the column using a gradient of 250 mM imidazole in the same buffer and the MSG protein eluted at ~90 mM imidazole. Protein in pooled fractions was unfolded (20 mM Tris, 100 mM NaCl, 10 mM 2-mercaptoethanol and 6 M guanidium chloride, pH 7.8) for 1 h at room temperature to allow full exchange of amide protons. Protein was refolded by rapid dilution (~1:50) into ice-cold refolding buffer (20 mM Tris, 100 mM NaCl, 10 mM 2-mercaptoethanol, 5 mM MgSO 4 , 10% sucrose and 6 cOmplete TM Mini Protease Inhibitor Cocktail tablets (Sigma) per litre buffer, pH 7.8). The protein was incubated, stirring at room temperature for 2 h before purification by affinity chromatography as described above. The pooled fractions were further purified by size-exclusion chromatography using a Superdex 200 5/150 gel filtration column (GE Healthcare) (20 mM NaPO 4 , 5 mM dithiothreitol) and the MSG eluted at ~75 mL. Overall, 20 mM MgCl 2 , 0.05% NaN 3 and 10% 2 H 2 O was added to the samples to make up the final NMR buffer. Database extractions The 13 C chemical shift distributions for arginine, isoleucine, valine, threonine, lysine and proline shown in Supplementary Fig. 1 were extracted from the BMRB database [20] using the PACSY database [34] and the provided API ( https://github.com/uwbmrb/BMRB-API ), which was embedded in an in-house written python script. NMR spectroscopy All 13 C-detected experiments were performed on a Bruker Avance II 600-MHz spectrometer using a 13 C-optimised TXO coldprobe or a Bruker Avance HD 800-MHz spectrometer using an HCN inverse TCI coldprobe equipped with cooled 1 H and 13 C preamplifiers. NMR experiments on T4L L99A The two-dimensional 13 C– 13 C correlation spectra in Fig. 2c , Supplementary Figs. 3 and 4 were all recorded at a static magnetic field of 14.1 T and a temperature of 278 K. The pulse sequence used was the one shown in Fig. 2a and Supplementary Fig. 2 . Deuterium 2 H decoupling was achieved using a constant-wave (CW) field applied at 1.1 kHz, which in our hands gave significantly better decoupling than using composite decoupling schemes, e.g. WALTZ16 [35] . During the INEPT transfers, the 2 H decoupling field was centred on the frequency of the 2 H bound to 13 C t , while for indirect chemical shift evolution, the 2 H decoupling field was centred on the frequency of the 2 H bound to 13 C p . For example, for arginine 13 C δ – 13 C γ , the 2 H decoupling field was centred at 1.55 ppm ( 2 H γ ) during the indirect chemical shift evolution and at 3.10 ppm elsewhere. Frequency-selective 90° (180°) pulses were applied with RE-BURP (E-BURP) [36] shapes. Spectra shown to the left (right) in Supplementary Figs. 2 and 3 were recorded with 10 (33) complex points in the indirect dimension, 4 scans per transient and a recovery delay of 4 s, leading to a total acquisition time of 12 min (38 min) per spectrum. The 13 C-detected CEST experiments were recorded at 14.1 T using the pulse sequence shown in Supplementary Fig. 9 . CEST experiments to characterise valine residues were recorded with 22 complex points in the 13 C β dimension (sweep width of 800 Hz) and 50 CEST saturation points between −600 and 600 Hz. Eight scans were recorded per transient and a recovery delay of 4 s was used, leading to a total acquisition time of 40 h. CEST experiments to characterise arginine and threonine residues were recorded with 30 complex points in the 13 C γ dimension (sweep width of 1136 Hz) and 42 CEST saturation points between −300 and 300 Hz. Sixteen scans were recorded per transient and a recovery delay of 4.4 s was used, leading to a total acquisition time of 98 h. The CEST field, ω CEST , and its inhomogeneity was obtained, as described by Guenneugues et al. [37] , using a 20 mM sample of [U- 2 H, 13 C]-isoleucine. Uncertainties in I / I 0 were estimated from duplicate measurements. The 3D long-range 13 C– 13 C scalar coupling experiment shown in Fig. 5a was recorded at 18.8 T and obtained using the pulse sequence shown in Supplementary Fig. 11 . The spectrum was recorded with 42 complex points in the indirect 13 C γ1 constant-time period ( t 2 ), 24 complex points in the indirect t 1 period, 8 scans per transient and a recovery delay of 4 s, leading to a total acquisition time of 75 h. Further experimental details are given in the legend of Supplementary Fig. 11 . NMR experiments on MSG The two-dimensional 13 C– 13 C correlation spectra in Fig. 1e and S8 were recorded at a static magnetic field of 18.8 T and a temperature of 310 K. The pulse sequence used was the one shown in Fig. 2a and Supplementary Fig. 2 . The two spectra in Fig. 3 were recorded with 43 complex points in the indirect constant-time dimension, 16 scans per transient and a recovery delay of 10 s, leading to a total acquisition time of 7.5 h per spectrum. The 3D 13 C– 13 C-TOCSY spectrum shown in Fig. 3b was recorded using the pulse sequence described in Supplementary Fig. 8 . The spectrum was recorded with 54 complex points in the indirect 13 C γ1 constant-time period ( t 2 ), 24 complex points in the indirect t 1 period, 4 scans per transient and a recovery delay of 10 s, leading to a total acquisition time of 120 h. Further experimental details are given in the legend to Supplementary Fig. 8 . The 3D long-range 13 C– 13 C scalar coupling experiment shown in Fig. 5b was obtained using the pulse sequence shown in Supplementary Fig. 11 . The spectrum was recorded with 42 complex points in the indirect 13 C γ1 constant-time period ( t 2 ), 27 complex points in the indirect t 1 period, 8 scans per transient and a recovery delay of 7.8 s, leading to a total acquisition time of 160 h. Further experimental details are given in the legend to Supplementary Fig. 11 . Chemical shift assignments The side-chain chemical shift assignment of T4L L99A was obtained based on the assignments published previously [6] , [11] combined with 1 H and 13 C-detected CC-TOCSY experiments and the 1 H and 13 C-detected long-range 3 J CαCδ experiments. The stereospecific assignment of the valine 13 C γ was taken from ref. [38] . The chemical shift assignment of the MSG valine 13 C γ – 13 C β correlation spectrum was transferred from a previously published assignment [26] , [27] , that in turn was based on 1 H-detected experiments. The chemical shift assignment of the isoleucine 13 C δ1 – 13 C γ1 spectrum was obtained by a combination of a previous assignment [26] , [27] and the 13 C-detected TOCSY experiment (Fig. 3b; Supplementary Fig. 8 ) and the 13 C-detected long-range 3 J CαCδ experiment (Fig. 5b; Supplementary Fig. 11 ). Data analysis All NMR spectra were processed using nmrPipe [39] and initially analysed using NMRFAM-Sparky [40] or CCPN [41] . Peak intensities in experiments reporting on relaxation rates and CEST, Fig. 4 and Supplementary Figs. 5 , 7 , 9 and 10 , were obtained using FuDA [42] , [43] . Long-range scalar couplings were derived by first obtaining the peak heights of the peaks corresponding to the diagonal peak, I d = I ( 13 C δ – 13 C γ – 13 C δ ) and the cross-peak I c = I ( 13 C α – 13 C γ – 13 C δ ) using the inbuilt tools of NMRFAM-Sparky and CCPN. The long-range scalar coupling was then calculated according to [4] I c / I d = tan [2] (2π J CC T J ), where J CC is the three-bond scalar coupling and T J is the coupling evolution delay in the pulse sequence in Supplementary Fig. 11 . As described previously [13] , passive couplings cancel by taking the ratio of I c and I d , such that this ratio only reports on the long-range coupling. For the 1 H-detected experiments, the error was determined as the root-mean-square deviation of two experiments. For the other long-range scalar coupling experiments, errors in the obtained I c and I d were estimated from RMSD of the spectral region, where no peaks were observed. The uncertainty of the calculated 3 J CC was estimated using a Monte-Carlo procedure to propagate the errors from the intensities. Carbon 13 C-detected CEST experiments were analysed using in-house written software in python using the LMFIT [44] module for least-squares minimisation of the target function 
    χ ^2(𝐩) = ∑_i ( Ĩ_obs,i - Ĩ_calc,i(𝐩))^2/σ ^2
 (1) where \(\tilde I_{{\mathrm{obs}},i}\) and σ are the experimentally obtained normalised intensities \(\left( {\tilde I = I/I_0} \right)\) and their uncertainty, respectively. The sum is over the different CEST saturation points and CEST field strengths, ω CEST . \(\tilde I_{{\mathrm{calc}},i}\) are the calculated normalised intentities calculated as a function of the model parameters p . Briefly, calculated intensities were obtained by evolving the spin system according to the Liouvillian described previously [14] , [19] , [45] , [46] , also taking into account the one-bond 13 C– 13 C scalar coupling, which generally leads to a simple line broadening of the CEST profiles. An inhomogeneity of the saturation field of 5% was used. The model parameters consist of the chemical shifts of the ground and excited states, ϖ G and ϖ E , respectively, the longitudinal relaxation rate that was assumed to be identical in the ground and excited state, R 1G = R 1E = R 1 and the transverse relaxation rate in the ground and excited states, R 1G , R 2E . For the analysis of R125, it was imposed that R 2G = R 2E , since the data did not contain enough information to determine R 2E ; for other fits, both R 2G and R 2E were determined. The overall exchange range, k ex , and the population of the excited state, p E , were treated as global parameters. Uncertainties of the obtained residue-specific parameters were estimated using the covariance method [47] , as implemented in LMFIT. The uncertainties of k ex and p E were estimated by performing a grid search (see Supplementary Fig. 10 ). Reporting summary Further information on research design is available in the Nature Research Reporting Summary linked to this article.